One-step synthesis of zero-dimensional hollow nanoporous gold nanoparticles with enhanced methanol electrooxidation performance Nanoporous gold with networks of interconnected ligaments and highly porous structure holds stimulating technological implications in fuel cell catalysis. Current syntheses of nanoporous gold mainly revolve around de-alloying approaches that are generally limited by stringent and harsh multistep protocols. Here we develop a one-step solution phase synthesis of zero-dimensional hollow nanoporous gold nanoparticles with tunable particle size (150–1,000 nm) and ligament thickness (21–54 nm). With faster mass diffusivity, excellent specific electroactive surface area and large density of highly active surface sites, our zero-dimensional nanoporous gold nanoparticles exhibit ~1.4 times enhanced catalytic activity and improved tolerance towards carbonaceous species, demonstrating their superiority over conventional nanoporous gold sheets. Detailed mechanistic study also reveals the crucial heteroepitaxial growth of gold on the surface of silver chloride templates, implying that our synthetic protocol is generic and may be extended to the synthesis of other nanoporous metals via different templates. Nanoporous gold structures are highly porous metallic structures characterized by their unique and comprehensive three-dimensional networks of nanoscale interconnected ligaments. These interconnected ligaments have curved surfaces dominated by highly active low-coordinated atoms, such as steps and kinks [1] , [2] , [3] , that serve as excellent catalytic sites for chemical reactions [4] , [5] , [6] , [7] . Owing to the extensive porous networks, the diffusivity within nanoporous gold is greatly enhanced, which facilitates the mass transfer of reactants from exterior surface to the interior structure, significantly enhancing the catalytic reactions even at low temperatures [8] , [9] . Hence, nanoporous gold structures have found potential applications in fuel cell, demonstrating remarkable catalytic activities towards various fuel cell reactions, such as oxidation of CO [10] , [11] , [12] , methanol [13] , ammonia borane [14] and hydrazine [15] . Currently, most nanoporous gold exists as two-dimensional (2D) sheet-like structures fabricated using methods such as de-alloying [16] , [17] , [18] , [19] , self assembly [20] , template [21] and electrochemical methods [22] . In particular, the de-alloying approach is the most frequently used protocols, which can also be extended to other nanoporous metals/alloys such as copper [23] , silver [24] , palladium [25] , platinum [26] , [27] , Pt-Ru [28] , Pd-Pt [29] , [30] and Pt-Au [31] . Erlebacher et al. [16] pioneered in de-alloying Au 32% Ag 68% sheets into thin nanoporous gold sheets, which exhibit characteristic 2D bicontinuous morphology and tunable pore size between 5 nm and 1 μm [17] . However, such de-alloying approach is limited by its prerequisite of >55 atomic% of silver to produce nanoporous gold effectively and also restricted to the formation of 2D thin film nanoporous gold with low surface area-to-volume ratio, which generally suffers from slow mass transfer of reactant and low density of catalytic sites [32] . Ideally, reducing the size of nanoporous gold to zero-dimensional (0D) nanoporous gold nanoparticle can further increase both its surface area-to-volume ratio and density of catalytic sites, boosting its catalytic performance over conventional 2D counterparts. Current synthesis of nanoporous gold nanoparticles still mainly revolves around the de-alloying approach. For instance, Wang and Schaaf [33] reported the synthesis of nanoporous gold nanoparticles by de-alloying composite nanoparticles formed via thermal de-wetting of Au-Ag bilayer. However, harsh reaction conditions, the need of at least 55 atomic% silver sacrificial template and the formation of polydisperse nanoparticles that are strictly substrate bounded greatly limit the practicality of such method for actual industrial application. While the reported catalytic activity of nanoporous gold has been promising, we envisage that a simple and cost-effective strategy to synthesize monodisperse free-standing nanoporous gold nanoparticle for superior catalytic performance is much needed to incorporate them to the existing membrane-based industrial fuel cell systems. Here, we report the solution-based, high-yield synthesis of free-standing hollow nanoporous gold nanoparticles with tunable particle and ligament sizes. We systematically characterize the morphology of our nanoporous gold nanoparticles and provide a detailed mechanistic study on the formation of such nanoparticles. Methanol electrooxidation activity, specific electroactive surface area and also tolerance towards carbonaceous species of various nanoporous gold nanoparticles is investigated thoroughly and their superiority over solid gold nanoparticles and conventional nanoporous gold sheets is demonstrated. The stability of our nanoporous gold nanoparticles is also evaluated over>400 catalytic cycles to demonstrate their potential suitability for future industrial applications. Synthesis of nanoporous gold nanoparticles We employ a one-step synthetic protocol to synthesize hollow nanoporous gold nanoparticles using HAuCl 4 as precursor, hydroquinone as reducing agent and polyvinylpyrrolidone (PVP) as surfactant in the presence of Ag + ions. In a typical synthesis, 160 μl of 28 mM hydroquinone solution, 60 μl of 10 mM AgNO 3 solution and 100 μl of 40 mM HAuCl 4 solution are added in sequence to a 4.5 ml of 90 mM PVP solution on gentle stirring at room temperature. The solution turns colorless immediately, changes to light green within the next 30 s and eventually to reddish in 3 min. After that, the solution is washed with concentrated NH 4 OH to remove residual AgCl formed during the reaction, and purified by repeated centrifugations and redispersal in water. Characterization of nanoporous gold nanoparticles Scanning electron microscope (SEM) image indicates that the as-synthesized nanoparticles are spherical in shape but exhibit highly roughened surface with randomly interconnected curved ligaments, which resembles ‘gyri’ ridges on human being’s brain ( Fig. 1a ). Typically, using the one-step synthesis, a yield of>90% can be produced with monodisperse nanoporous gold nanoparticle sizes of (150±10) nm. A close inspection reveals a large number of nano-sized gaps in between the ligaments on the nanoparticles ( Fig. 1b ). The surface texture of our nanoparticles is analogous to the 2D nanoporous gold film made by de-alloying method [16] . To the best of our knowledge, this is the first report on using solution-based approach to synthesize free-standing nanoporous gold nanoparticles. From here onwards, we will refer these particles as ‘np-Au 150’, where ‘np-Au’ and the following number denote to ‘nanoporous gold nanoparticles’ and their corresponding size in nanometer length scale, respectively. It is noteworthy that, comparing with conventional gold nanoparticles, our as-synthesized particles are highly porous in morphology. The reason for the formation of such porous structures will be discussed in details in the mechanism section. The nanoporous gold with anisotropic morphology is expected to have a high surface area, which is particularly crucial for catalytic applications. 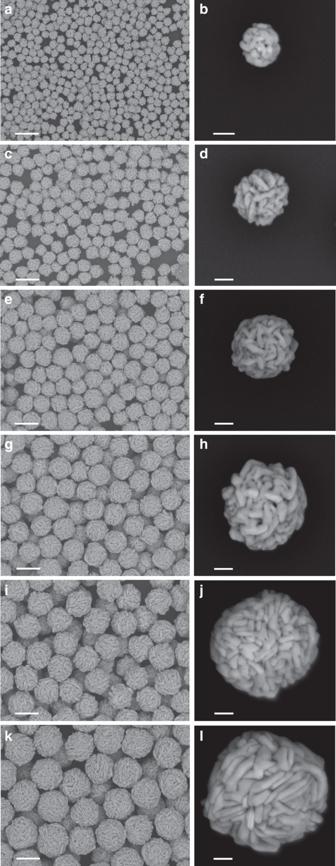Figure 1: Structural characterization of nanoporous gold nanoparticles. SEM images of various sized nanoporous gold nanoparticles (np-Au): (a,b) 150 nm, (c,d) 250 nm, (e,f) 350 nm, (g,h) 450 nm, (i,j) 550 nm and (k,l) 650 nm in diameter. The size is tuned by varying the final concentration of hydroquinone from 0.4 mM to 1.3 mM while maintaining all other conditions during the synthesis. (a,c,e,g,i,k) Scale bars, 500 nm. (b,d,f,h,j,l) Scale bars, 100 nm. Figure 1: Structural characterization of nanoporous gold nanoparticles. SEM images of various sized nanoporous gold nanoparticles (np-Au): ( a , b ) 150 nm, ( c , d ) 250 nm, ( e , f ) 350 nm, ( g , h ) 450 nm, ( i , j ) 550 nm and ( k , l ) 650 nm in diameter. The size is tuned by varying the final concentration of hydroquinone from 0.4 mM to 1.3 mM while maintaining all other conditions during the synthesis. ( a , c , e , g , i , k ) Scale bars, 500 nm. ( b , d , f , h , j , l ) Scale bars, 100 nm. Full size image The size of the nanoporous gold nanoparticles can be systematically controlled by varying the concentration of the reducing agent, hydroquinone. With increase in the final concentration of hydroquinone from 0.6 mM, 0.8 mM, 1 mM and 1.3 mM, nanoporous gold particles with increasing average sizes of (246±15) nm ( Fig. 1c,d ), (350±16) nm ( Fig. 1e,f ), (448±18) nm ( Fig. 1g,h ) and (550±14) nm ( Fig. 1i,j ), respectively, are observed. We also notice the ligament thickness increases with the size of the nanoporous particles, that is, from (21±3) nm to (51±8) nm for np-Au 150 and np-Au 550, respectively ( Table 1 ). Larger nanoporous gold particle in the range of 650–1,000 nm can be achieved by further increasing the concentration of hydroquinone and gold precursor used ( Supplementary Fig. 1 ). For instance, np-Au 650 ( Fig. 1k,l ) with a ligament size of (54±9) nm is synthesized by doubling the amount of hydroquinone and gold precursor added during the synthesis. Table 1 Summary of the structural and electrochemical properties of nanoporous gold nanoparticles. Full size table We investigate the internal structure of nanoporous gold nanoparticles by sectioning the nanoporous gold using ultracut-microtome. Nanoparticles are casted in an epoxy, and sliced into a 100-nm thin section. 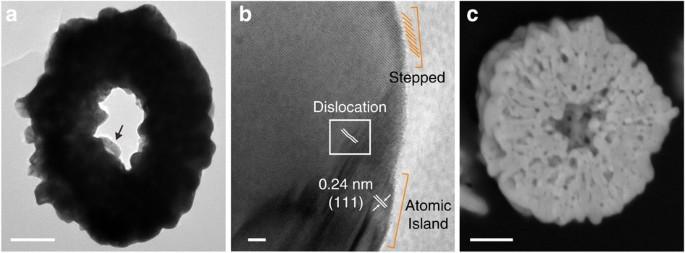Figure 2: Internal structure of nanoporous gold nanoparticles using electron microscopy characterization. (a) TEM image of a microtome-sectioned np-Au 550; the arrow indicates a free-standing ligament. (b) High-resolution TEM image of a single ligament indicating the presence of step feature, dislocation and atomic island. (c) Cross-sectional SEM image of a microtome-sectioned np-Au 550 nm. (a,c) Scale bars, 100 nm. (b) Scale bar, 2 nm. Figure 2a shows a general morphology of microtome section of nanoporous gold nanoparticles of size 550 nm, which clearly indicates the formation of a hollow nanoparticle. The periphery of the nanoporous gold exhibits undulating curvatures and highly roughened surfaces, with occasional ligament protruding freely from the main body (see arrow in Fig. 2a ). Figure 2: Internal structure of nanoporous gold nanoparticles using electron microscopy characterization. ( a ) TEM image of a microtome-sectioned np-Au 550; the arrow indicates a free-standing ligament. ( b ) High-resolution TEM image of a single ligament indicating the presence of step feature, dislocation and atomic island. ( c ) Cross-sectional SEM image of a microtome-sectioned np-Au 550 nm. ( a , c ) Scale bars, 100 nm. ( b ) Scale bar, 2 nm. Full size image High-resolution transmission electron microscopy (TEM) image of a ligament offers insights into the atomic arrangement and morphology of the nanoporous gold nanoparticles. In general, the ligaments possess concave surfaces with high crystallinity. Characteristic lattice fringes are observed over the whole ligament. A d-spacing of 2.4 Å corresponding to face-centered cubic (fcc) Au (111) facet is measured ( Fig. 2b ), indicating that (111) is the mostly exposed plane. Using the high-resolution TEM images obtained ( Supplementary Fig. 2 ), we determine an average crystallite size of (16.9±4.2) nm for np-Au 550. A significant feature of ligament is that there are many zig-zag features on the exterior of the ligament, demonstrating the presence of high density of atomic defects. For example, we observe (111) terraces separated by atomic steps, which are probably stabilized by the trace amount of Ag along the edges of the ligaments [2] . In addition, we observe atomic layer islands ( Fig. 2b ) on the surface of the ligaments. It has been reported that the presence of high-density atomic defects such as steps and kinks is the basis for the origin of high catalytic activity in gold catalyst [2] , [3] , [4] . Similarly, the presence of these features in our nanoporous gold nanoparticles may aid the enhancement of the catalytic performance. Furthermore, the high-resolution SEM image of microtome-sectioned np-Au 550 demonstrates the entire body of our nanoporous gold is formed entirely by interconnected ligaments ( Fig. 2c ), with 3D porous network of pore size ranging from 3 to 30 nm. A hole is visible at the centre of the particle, demonstrating its hollow interior. Similar hollow interior is also confirmed on focused ion beam milled nanoporous gold nanoparticle ( Supplementary Fig. 3 ). The selected area electron diffraction pattern of np-Au 550 ( Supplementary Fig. 2f ) consists of a combination of diffraction spots and ring structure, indicating that the entire particle is nanocrystalline in nature. The ring patterns in selected area electron diffraction pattern reveal the randomly oriented crystallites and are characteristic of polycrystalline gold [35] . To resolve the crystallinity and structure of the bulk nanoporous gold nanoparticles, powder X-ray diffraction (XRD) is employed. The XRD spectra for np-Au 150, 250, 350, 450, 550 are compared with the solid gold nanoparticles of size 200 nm ( Supplementary Fig. 4 ). Five sharp diffraction peaks are observed for all the six samples at 38.3°, 44.5°, 64.7°, 77.7° and 81.9° in the 2θ range of 20–85°, which are indexed to the {111}, {200}, {220}, {311} and {222} reflections ( Supplementary Table 1 ) of fcc phase of metallic gold (JCPDS, card No. 04-0784). Among all, the diffraction peak corresponding to the {111} plane at 38.3° is the most intense, which can be attributed to the large exposed area of the corresponding facets, whereas the remaining less intense peaks are associated to the less-exposed facets. The relative intensities of diffraction peaks for all six samples differ with standard powder diffraction data. The intensity ratio of {200}:{111} diffraction is 0.34 for the as-prepared nanoporous gold nanoparticles ( Supplementary Table 2 ), which is smaller than the 0.52 intensity ratio of the standard Au diffraction database. The result indicates our nanoporous gold nanoparticles exhibit a preferred orientation along the {111} plane, whereas solid gold nanoparticles demonstrate random growth due to the differences in multiple relative intensities compared with standard Au data. In addition, the mean crystallite size is also calculated using Scherrer equation owing to its influence on the properties of the metals, including strength and hardness. We would like to emphasize that although Scherrer equation is largely based on cubic crystal model, the crystallite shape factor can be approximated to 0.9 in absence of shape information [36] , [37] . 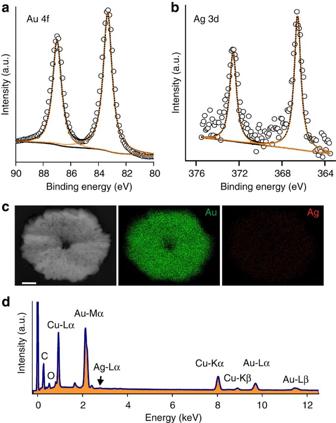Figure 3: Elemental composition and distribution of nanoporous gold nanoparticles. X-ray photoelectron spectroscopic analysis of np-Au 150 at (a) Au 4f and (b) Ag 3d binding energy windows, respectively. (c) EDS elemental mapping of a microtome-sectioned nanoporous gold nanoparticles indicating the Au and Ag elemental distribution, and (d) the corresponding EDS elemental spectrum of np-Au 550. (c) Scale bars for all, 100 nm. Using Scherrer equation and the full-width half maximum of the XRD peak at {111} plane [38] , the mean crystallite sizes are estimated at 13.1, 14.8, 14.8, 14.6 and 14.6 nm for np-Au 150–550, respectively ( Supplementary Table 3 ), consistent with the thickness of the ligaments measured from high-resolution TEM ( Fig. 2a and Supplementary Fig. 2 ). Elemental composition and distribution of np-Au particles X-ray photoelectron spectroscopy (XPS) is used to determine the surface composition, both in terms of elements and oxidation states, of the as-synthesized nanoporous gold nanoparticles. The high-resolution Au 4f scan ( Fig. 3a ) for np-Au 150 reveals a doublet at 87.2 and 83.5 eV separated by~3.7 eV, confirming the presence of zero-valent gold in nanoporous gold nanoparticles. The high-resolution Ag 3d scan ( Fig. 3b ) indicates two weak binding energy peaks at 373.5 eV and 367.5 eV, which can be attributed to the spin-orbital splitting of Ag3d 3/2 and Ag3d 5/2 electron states with intensity ratio of 2:3. This confirms the presence of silver in its elemental form. Based on the XPS results, an atomic ratio of 95:5 for Au:Ag is measured, affirming that nanoporous gold nanoparticles are mostly made from gold with trace amount of silver. The atomic percentage of silver decreases from the initial stoichiometric of 13 to 5% may be due to the removal of silver entity from the final product, probably as silver chloride. Figure 3: Elemental composition and distribution of nanoporous gold nanoparticles. X-ray photoelectron spectroscopic analysis of np-Au 150 at ( a ) Au 4f and ( b ) Ag 3d binding energy windows, respectively. ( c ) EDS elemental mapping of a microtome-sectioned nanoporous gold nanoparticles indicating the Au and Ag elemental distribution, and ( d ) the corresponding EDS elemental spectrum of np-Au 550. ( c ) Scale bars for all, 100 nm. Full size image We also perform energy-dispersive X-ray spectroscopy (EDS) analyses to determine the distributions of gold and silver in the microtome section of np-Au 550 nm. The Au and Ag EDS maps are acquired from the peaks at 2.1 and 2.9 keV ( Fig. 3d ), which can be assigned to Au Mα and Ag Lα, respectively. The EDS mapping ( Fig. 3c ) clearly shows that gold is homogenously distributed on the whole surface of np-Au 550, whereas only trace amount of silver is present, which could be used to stabilize the curved surfaces [39] . EDS elemental spectra ( Fig. 3d ) further confirms that the np-Au 550 is predominantly gold (99 atomic%) with residual silver (1 atomic%). From the higher silver percentage measured using XPS, we therefore suggest that silver is predominantly present on the nanoparticle surfaces to stabilize the low-coordinated gold atoms because XPS is a surface sensitive technique, whereas EDS of a cross-sectioned nanoporous gold measures the overall silver percentage. Mechanistic study on the formation np-Au To better understand the formation process of nanoporous gold nanoparticles, we monitor the evolution of the morphology of the nanocrystals over time ( Fig. 4 and Supplementary Fig. 5 ). In the absence of hydroquinone, the addition of AgNO 3 and HAuCl 4 to PVP solution results in a color change from yellowish to whitish yellow (inset of Supplementary Fig. 5a ), indicating a reaction has taken place. From SEM, particles with cubic morphology of an approximate average size of 230 nm are observed ( Supplementary Fig. 5a ). These cubic particles are highly unstable and tend to decompose under electron beam. The reaction is hypothesized to be: AuCl 4 − +4 Ag + → Au 3+ +4 AgCl. Our hypothesis is confirmed by the XPS elemental composition measurement of these particles which clearly indicates the presence of Ag + and Cl − ( Supplementary Fig. 5a ). We also note a smaller doublet presents in the Ag scan, which is attributed to the presence of metallic silver due to the photoreduction of Ag + → Ag 0 under electron beam. On the addition of 20 μl of hydroquinone into the above reaction mixture, nucleation of asymmetric (plate-like and spherical shape) particles onto the AgCl nanocrystals are observed ( Fig. 4d ). These particles are identified as metallic gold nanoparticles with atomic ratio of Au:Ag + of 2:98 (as evident from XPS results in Supplementary Fig. 5b and 5e ). We do not observe the formation of individual gold nanoparticles. This is probably because the heterogeneous growth of gold on the pre-formed AgCl seeds is energetically more favorable than the homogeneous nucleation of gold nanoparticles [40] . 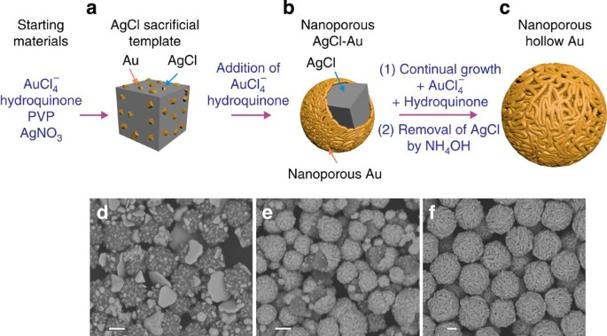Figure 4: Mechanism of nanoporous gold nanoparticles formation. (a–c) A schematic synthetic route for the formation of hollow nanoporous gold nanoparticles using AgCl as sacrificial template. (d–f) The representative SEM images obtained at the corresponding stages during the formation of nanoporous gold nanoparticles. (d–f) Scale bars, 200 nm. Figure 4: Mechanism of nanoporous gold nanoparticles formation. ( a – c ) A schematic synthetic route for the formation of hollow nanoporous gold nanoparticles using AgCl as sacrificial template. ( d – f ) The representative SEM images obtained at the corresponding stages during the formation of nanoporous gold nanoparticles. ( d – f ) Scale bars, 200 nm. Full size image Further increasing the amount of hydroquinone leads to continual growth of gold on AgCl sacrificial template. In the meantime, the aqueous phase color gradually turns red (inset of Supplementary Fig. 5c ). In addition, the originally asymmetric nanoparticles are transformed into ligament structures, indicating Ostwald ripening has occurred on further addition of reducing agent ( Fig. 4e ). Correspondingly, the atomic ratio of Au:Ag + also increases to 90:10 ( Supplementary Fig. 5c,e ). After treating the nanoparticle solution with NH 4 OH solution, we observe a cavity of size about 200 nm at the centre of the particles ( Supplementary Fig. 5d ), which is consistent with the width of AgCl template (~200 nm).The result therefore clearly demonstrates that AgCl sacrificial template can be easily removed to form the hollow nanoporous gold nanoparticles ( Fig. 4f ). This observation is further confirmed by a decrease in Ag° to 5 atomic%, giving an overall Au:Ag ratio of 95:5 as quantified using XPS ( Fig. 3a,b ). Electrochemical performance of np-Au versus solid particles The facets on the curved ligaments on our nanoporous gold nanoparticles contain high density of low-coordinated atoms ( Fig. 2b ), which are ideal catalytically active sites. In the following sections, we perform electrooxidation of methanol as a model reaction to examine the catalytic activity of our nanoporous gold nanoparticles. We begin by comparing the cyclic voltammetry (CV) of np-Au 250 nanoparticles with solid gold nanoparticles of ~250 nm and 30 nm, which are denoted as Au 250 and Au 30 from now onwards, in 2 M methanol and 0.5 M KOH solution ( Fig. 5a ). The Au 250 resembles the macroscopic size of np-Au 250, whereas Au 30 resembles the ligament size of the np-Au 250. 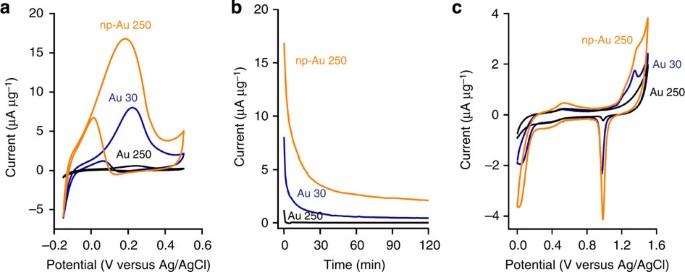Figure 5: Electrochemical performance of nanoporous versus solid gold nanoparticles. The catalytic methanol electrooxidation measurements in the form of (a) cyclic voltammograms and (b) chronoamperograms of np-Au 250, solid Au 30 and solid Au 250 nanoparticles in deoxygenated solution of 0.5 M KOH and 2 M CH3OH. The chronoamperograms were collected at the peak methanol oxidation of the corresponding nanoparticles, that is, 0.19 V, 0.22 V and 0.25 V for 120 min for np-Au 250, solid Au 30 and solid Au 250 modified electrodes, respectively. (c) Oxide stripping curves of the np-Au 250, solid Au 30 and solid Au 250 modified electrodes at a scan rate of 5 mV s−1in 0.5 M H2SO4electrolyte. Figure 5: Electrochemical performance of nanoporous versus solid gold nanoparticles. The catalytic methanol electrooxidation measurements in the form of ( a ) cyclic voltammograms and ( b ) chronoamperograms of np-Au 250, solid Au 30 and solid Au 250 nanoparticles in deoxygenated solution of 0.5 M KOH and 2 M CH 3 OH. The chronoamperograms were collected at the peak methanol oxidation of the corresponding nanoparticles, that is, 0.19 V, 0.22 V and 0.25 V for 120 min for np-Au 250, solid Au 30 and solid Au 250 modified electrodes, respectively. ( c ) Oxide stripping curves of the np-Au 250, solid Au 30 and solid Au 250 modified electrodes at a scan rate of 5 mV s −1 in 0.5 M H 2 SO 4 electrolyte. Full size image In the presence of 2 M methanol in 0.5 M KOH solution, np-Au 250, solid Au 30 and solid Au 250 nanoparticles exhibit the characteristic methanol electrooxidation behavior. For np-Au 250, an instant surge in current is observed from −0.15 V (versus Ag/AgCl) onwards in positive potential scan ( Fig. 5a ). It peaks at 0.19 V, and reaches a maximum current of 16.8 μA μg −1 , which corresponds to the oxidation peak of methanol [41] . In the negative sweeping scan, the reduction peak is observed 0.14 V, indicating the reduction of Au-OH species to Au. A second oxidation peak observed at 0.01 V in the reverse scan is attributed to the removal of the incompletely oxidized carbonaceous species formed in the forward scan [41] . On the other hand, solid Au 30 and Au 250 nanoparticles exhibit much reduced methanol oxidation peak with current of 8 μA μg −1 and 0.6 μA μg −1 , at relatively higher oxidation potentials of 0.22 V and 0.25 V, respectively. The respective gold oxide reduction peaks of Au 30 and Au 250 are observed at 0.16 V and 0.20 V. This result indicates our nanoporous gold nanoparticles exhibit a 2 and 28 times more superior catalytic activity towards methanol oxidation as compared with its solid counterparts. Such enhanced electrochemical activity of our nanoporous gold nanoparticles is remarkable, especially when comparing with solid gold nanoparticles of 30 nm whose size is equivalent to the ligament’s dimension. In addition, on the basis of electrooxidation of methanol (1 M) under alkaline media (0.5 M KOH), our np-Au 250 exhibits 1.4 times higher catalytic activity (117 μA cm −2 ) and improved tolerance towards carbonaceous species ( I f / I b =2.5) when compared with conventional nanoporous gold sheets (88 μA cm −2 and I f / I b =3) ( Supplementary Fig. 6b ) [42] . We attribute the superior catalytic performance of our nanoporous gold to the high density of highly active low-coordinated atoms present on the interconnected network of ligaments, which are densely distributed over the entire hollow spherical nanoparticles. Furthermore, the highly porous network of ligaments and large surface area-to-volume ratio of 0D nanoparticles facilitates the diffusion and mass transfer of electrolyte to the catalytically active surface for reaction. To affirm that the high electroactivity and characteristic oxidation peak are due to nanoporous gold nanoparticles and oxidation of methanol respectively, we conduct similar CV studies in the absence of methanol and in blank glassy carbon electrode. In the absence of methanol, the CV of np-Au 250 exhibits a single broad oxidation peak in the potential range between+0.30 to 0.50 V, indicating the formation of surface Au oxide by the adsorption of OH − ions (blue trace, Supplementary Fig. 6 ). In the negative sweeping scan, a reduction peak at 0.05 V, corresponding to Au oxide reduction is observed [43] . When using glass carbon-only electrode, no characteristic oxidation peak is observed even in the presence of methanol (black trace, Supplementary Fig. 6 ), indicating that the catalytic electrooxidation effect is solely originating from the nanoporous gold nanoparticles (orange trace, Supplementary Fig. 6 ). One of the problems concerning the catalytic methanol electrooxidation is the adsorption of poisoning intermediate carbonaceous species on catalysts’ surfaces [44] , [45] , which will deactivate the catalysts’ surface from further oxidation. The catalyst tolerance to the poisoning species in gold is often evaluated using the ratio of the forward anodic peak current ( I f ) to the backward anodic peak current ( I b ) [44] . A high I f / I b value signifies poor capability of catalyst to remove incompletely oxidized carbon species from the surface. On the contrary, a lower I f / I b value indicates the improved performance to eliminate residual carbon species via oxidation in the reverse scan. Our np-Au 250 is observed to have the lowest I f / I b of 2.5, as compared with 6.7 and 9.4 of Au 30 and Au 250 ( Fig. 5a ), respectively. Thus, np-Au 250 is expected to eliminate residual carbon species more readily and have prolonged electrocatalytic performance in comparison with solid Au 30 and Au 250. To evaluate the long-term electrocatalytic performance and tolerance of nanoporous gold catalysts, we study the chronoamperograms of the np-Au 250, solid Au 250 and Au 30. The current–time response of the np-Au 250, Au 30 and Au 250 are recorded at a 0.19 V, 0.22 V and 0.25 V, which correspond to their respective peak oxidative potentials ( Fig. 5b ). np-Au 250 exhibits a gradual decrease in current, reaching steady state at 2.6 μA μg −1 after 60 min, whereas the currents of solid Au 30 and Au 250 nanoparticles decrease exponentially and diminish to 0.5 and 0 μA μg −1 after 60 min. The rapid decreases of the current in Au 30 and Au 250 is mainly due to the higher tendency for the accumulation of carbonaceous intermediates that deactivates catalytic sites, as observed from their respective high I f / I b values of 6.7 and 9.4 determined previously. Hence, both the comparison of chronoamperometry and I f / I b ratio collectively exemplify the superior stability and activity of our np-Au 250 nanoparticles as a catalyst over solid gold nanoparticles. The electrochemical active surface area of np-Au 250, solid Au 30 and Au 250 nanoparticles are estimated by performing an electrochemical gold oxide stripping reaction in 0.5 M H 2 SO 4 aqueous solution at a scan rate of 5 mV s −1 in room temperature ( Fig. 5c ). The nanoporous gold nanoparticles exhibit a lower oxidation peak around 1.1 V as compared with solid Au 30 and Au 250 nanoparticles (1.2 V), indicating that surface atoms on our nanoporous gold nanoparticles are easier to oxidize. From these CVs, we estimate the electrochemically active surface areas by integrating the area of the gold oxide reduction curve near 0.9 V and assuming a specific charge of 450 μC cm −2 for the gold oxide reduction [46] . Electroactive surface areas of 8.91, 4.80 and 0.25 m 2 g −1 are obtained for np-Au 250, solid Au 30 and Au 250 catalysts, respectively ( Table 1 ). That is, our nanoporous gold nanoparticles are able to provide at least 2 and 36 times higher specific electroactive surface area for catalysis as compared with solid Au 30 and Au 250 nanoparticles, respectively. The superiority of our np-Au 250 is therefore a clear demonstration on the necessity of both nanoporosity and also large and extensive network of nanoscale ligaments, with high density of low-coordinated active surface Au atoms, to provide large electroactive surface area ( Fig. 2b ). Size-dependent electrochemical performance of np-Au In the following section, the size-dependent methanol oxidation of nanoporous gold nanoparticles of size ranges from 150–550 nm are performed ( Fig. 6a , Supplementary Table 4 ). A clear size dependency of maximum current and the onset potential are observed for nanoporous gold nanoparticles of all sizes. In the oxidative scan, a negative shift in onset potential from −0.12 V to −0.13 V is observed with decreasing nanoporous gold particles size from 550 to 150 nm ( Fig. 6b ). Earlier onset potential of 0.01 V observed in np-Au 150, when compared with np-Au 550, indicates that methanol is easier to be oxidized on nanoporous gold particles of smaller sizes, which we attribute to the higher electroactive surface area available in np-Au 150. The greater ease of methanol oxidation on small nanoparticle sizes is again supported by the 1.2 times higher peak methanol oxidation current, a parameter indicative of reaction rate, using np-Au 150 (17 μA μg −1 ) than that of np-Au 550 (15 μA μg −1 , Fig. 6c ). Furthermore, during a reduction scan, we observe a shift of the Au-OH reduction peak at 0.13 V to 0.17 V and also a decrease of current from −0.7 μA μg −1 to −0.3 μA μg −1 when particle sizes increase from np-Au 150 to np-Au 550. The reduced Au-OH reduction peak current with particle sizes indicates a decrease in the extent of Au-OH to Au conversion, which can be explained by the higher coverage of hydroxide species on np-Au 150 as a consequence of larger electroactive surface area present when compared with np-Au 550. We would like to emphasize that mass-normalized current is discussed instead of surface area-normalized currents to clearly exemplify the importance of high specific electroactive surface area and large mass diffusivity associated with smaller 0D nanoporous gold nanoparticles (refer to Supplementary Fig. 7c for detailed illustration). 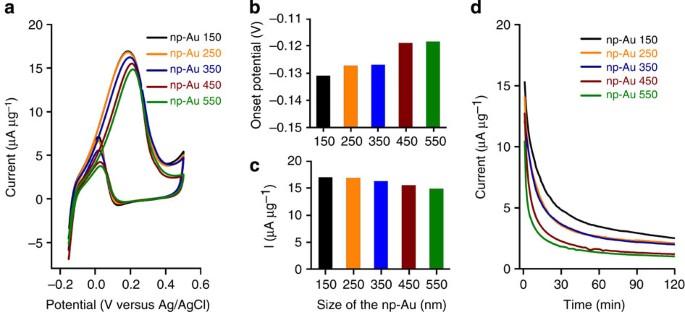Figure 6: Size-dependent electrochemical performance of nanoporous gold nanoparticles. Comparison of (a) cyclic voltammograms, (b) onset potential and (c) peak methanol oxidation current activity of nanoporous gold nanoparticles size from 150 nm to 550 nm. The methanol oxidation reactions were performed at a scan rate of 20 mV s−1in deoxygenated solutions with 0.5 M KOH and 2 M CH3OH. (d) Chronoamperograms of np-Au 150–550 modified electrodes at their corresponding peak oxidation potentials for 120 min. Figure 6: Size-dependent electrochemical performance of nanoporous gold nanoparticles. Comparison of ( a ) cyclic voltammograms, ( b ) onset potential and ( c ) peak methanol oxidation current activity of nanoporous gold nanoparticles size from 150 nm to 550 nm. The methanol oxidation reactions were performed at a scan rate of 20 mV s −1 in deoxygenated solutions with 0.5 M KOH and 2 M CH 3 OH. ( d ) Chronoamperograms of np-Au 150–550 modified electrodes at their corresponding peak oxidation potentials for 120 min. Full size image To investigate the size-dependent long-term electrocatalytic performance and tolerance of nanoporous gold catalysts in methanol oxidation reaction, we monitor the chronoamperograms of the np-Au 150–550 nm at their oxidation potentials for 2 h ( Fig. 6d , Supplementary Table 5 ). In general, the current for methanol oxidation shows a gradual decay during first 25 min, attributed to the accumulation of poisonous intermediate species before reaching a steady state after 60 min [47] . Particularly, the np-Au 150 modified electrode exhibits the highest initial current and slowest current decay compared with electrodes using nanoporous gold nanoparticles of larger size. In addition, the oxidation current of np-Au 150 is noticeably higher (2.52 μA μg −1 ) than other sizes even after extended reaction duration of 2 h. Hence, the results indicate a better tolerance and stability of np-Au 150 towards methanol oxidation reaction compared with larger nanoparticle sizes. The superior stability of np-Au 150 is again supported by its I f / I b ratio of 2.4, which is the lowest among all the nanoparticle sizes analyzed ( Supplementary Table 4 ) and also an indication of improved tolerance towards residual carbon species compared with commercial Pt/C catalyst [44] . The electrochemical active surface areas of various sized nanoporous gold nanoparticles are estimated by performing electrochemical gold oxide stripping reactions ( Supplementary Fig. 8 ). Our nanoporous gold nanoparticles typically exhibit a constant oxidation peak around 1.1 V for all particle sizes and the corresponding electroactive surface areas for np-Au 150, 250, 350, 450 and 550 nm catalysts are calculated at 9.1 , 8.9, 7.7, 7.3 and 6.8 m 2 g −1 , respectively ( Table 1 ). The oxidation peak potential using our nanoporous gold nanoparticles is lower compared with reported concave gold nanocubes (1.2 V) [48] , tetrahexahedral gold nanoparticles (1.18 V) and octahedral gold nanoparticles (1.35 V) [49] , indicating that surface atoms on our nanoporous gold nanoparticles are easier to oxidize and hence more catalytically active. It is also noted that all our nanoporous gold nanoparticles exhibit higher electroactive surface compared with 2D nanoporous gold sheets (6.4 m 2 g −1 ) [46] , with our best-performing np-Au 150 demonstrating at least 1.4-fold higher catalytic surface area. That is, our np-Au 150 can potentially provide at least 1.4-fold improved electrocatalytic performance compared with 2D nanoporous gold sheets fabricated via de-alloying approach, emphasizing the importance of 0D particles, and the presence of hollow interiors and porous surfaces for enhanced catalytic activities. To meet the requirements for actual fuel cell applications, we also evaluate the stability of our best-performing np-Au 150 through multiple electrocatalytic cycles of methanol oxidation. np-Au 150 exhibits highly stable current over 100 and 480 cycles, with the retention of at least 95 and 64% of electrocatalytic performance, respectively ( Supplementary Fig. 9 ). It is noteworthy that no obvious change in morphology is observed for the first 100 cycles ( Supplementary Fig. 10b and Supplementary Fig. 11 ). The ligaments on the surface only starts to appear coarsened and smoothened after an extended 480 electrocatalytic cycles, which is potentially the cause of the observed decrease of electrocatalytic performance from 95 to 64% ( Supplementary Fig. 10c ). Nevertheless, the highly reproducible and superior electrocatalytic performance of our nanoporous gold nanoparticles, together with the ease of incorporation to existing membrane-based fuel cell systems, will enable it as an attractive candidate for actual fuel cell application. We have developed a synthetic approach to synthesize 0D hollow nanoporous gold nanoparticles through a novel one-step solution phase method at room temperature. The mean size of our nanoporous gold nanoparticles can be systematically controlled between 150–1,000 nm by varying the concentration of hydroquinone. Using high-resolution transmission electron microscopy, we identify the presence of high density of steps and kinks along the curved surface on the ligaments, whose width can be in turn tailored between 21±3 and 51±9 nm. The formation process for the nanoporous gold is studied in detail using SEM and high-resolution XPS, with the critical step for the formation of nanoporous gold being the heteroepitaxial growth of Au on the surface of AgCl. The importance of small 0D nanoporous nanoparticles is clearly demonstrated by the enhanced electrocatalytic performance and improved tolerance to carbonaceous species during methanol oxidation with the decrease of the size of nanoporous gold nanoparticles. Our nanoporous gold nanoparticles exhibit at least 1.4 times higher catalytic activity compared with conventional solid gold nanoparticles and existing nanoporous gold sheets. Our synthetic protocol is also generic and can be extended to different templates to further tailor the thickness of ligament, porosity and ultimately, enhancing catalytic activities. With the ensemble of benefits, our nanoporous gold nanoparticles and synthetic methodology are expected to have a strong impact in the area of fuel cell development, where scalable synthesis, high catalytic performance and easy transition from lab-based system to industrial application are crucial. Materials Silver nitrate (99+ %), poly(vinyl pyrrolidone) (PVP, M w =1,300 K), hydroquinone (≥99%), L -ascorbic acid (99%), hydroxylamine hydrochloride (99.99%), and gold(III) chloride trihydrate (≥99.9%) and were purchased from Sigma-Aldrich; ammonia solution was obtained from Goodrich Chemical Enterprise; ethanol (ACS, ISO, Reag.) and methanol were purchased from EMSURE. All chemicals were used without further purification. Milli-Q water (> 18.0 MΩ cm) was purified with a Sartorius arium611 UV ultrapure water system. Synthesis of hollow nanoporous gold nanoparticles In sequence, 160 μl of 28 mM hydroquinone solution, 60 μl of 10 mM AgNO 3 solution and 100 μl of 40 mM HAuCl 4 solution were added to 4.5 ml of 90 mM PVP solution on gentle stirring at room temperature. Nanoporous gold nanoparticles from 250 to 550 nm are synthesized by increasing the final concentration of hydroquinone from 0.6–1.3 mM respectively. The mixture was kept stirring for 3 min as the color of the solution changed from colorless to greenish to reddish brown. The solution was kept undisturbed for 30 min. After that, the solution is washed with concentrated NH 4 OH to remove residual AgCl formed during the reaction, and purified by repeated centrifugations at 5,000 r.p.m. for 5 min and re-dispersal in water. Synthesis of solid 30-nm gold nanoparticles A quantity of 0.5 ml of ascorbic acid (28 mM) was added to an aqueous solution containing 180 mM PVP and 0.5 mM HAuCl 4 on rigorous stirring. The color of the solution turned from colorless to red immediately indicating the formation of nanoparticles. Synthesis of solid 200-nm gold nanoparticles 200-nm gold nanoparticles was prepared through the one-step seed-mediated process using 30-nm gold seeds. Briefly, 100 μl of the as-synthesized 30 nm seed particles was added to a 10 ml growth solution containing 55 mM CTAB, 25 mM HAuCl 4 and 4 mM ascorbic acid. The solution was kept undisturbed for 1 h at room temperature. The product was then collected by centrifugation at 6,000 r.p.m. for 5 min. Measurement of particle size The sizes of the nanoporous gold nanoparticles were analyzed on the basis of SEM images using Nano Measurer analysis software (Department of Chemistry, Fudan University, China). The histograms were plotted by measuring at least 100 particles. Piranha treatment of nanoporous gold nanoparticles Nanoporous gold nanoparticles are treated with piranha solution (3:1 mixture of concentrated H 2 SO 4 and 30% H 2 O 2 ) to remove the PVP on the surface of the nanoparticles. Briefly, 5 ml of piranha solution was added to the aqueous solution containing nanoporous gold nanoparticles and solution was undisturbed for 30 min before centrifugation at 6,000 r.p.m. for 5 min. The particles were further washed three times to remove trace amounts of acid and re-dispersed in ethanol followed by vacuum drying to collect the nanoporous gold particles before conducting of the electrochemical measurements. Nanoporous gold modified electrode preparation A quantity of 1 mg of nanoporous gold sample was suspended in a solution containing 1 ml ethanol by ultrasonication. A quantity of 1 μl of the suspension was drop-casted on glassy carbon electrode surface. The electrode was air dried for 1 h at room temperature before use. Electrochemical measurements Electrochemical measurements were carried out using Metrohm Auto lab potentiostat instrument. Three electrodes configuration was employed. The working electrode used was nanoporous gold nanoparticles modified glassy carbon electrode, a leak-free saturated Ag/AgCl electrode as reference and the counter electrode was a Pt wire. A quantity of 0.5 M KOH solution was used as an electrolyte. Estimation of electrochemical surface area The electrochemical active surface area of various sized nanoporous gold nanoparticles and solid Au nanoparticles were estimated using CV. The surface redox behavior of the nanoporous gold nanoparticles and solid Au nanoparticles were characterized using CV in 0.5 M H 2 SO 4 aqueous solution at a scan rate of 5 mV s −1 in room temperature. The electrochemical active surface area is estimated from the equation of Q o =2eNAΓ o A, where Q o is the charge passed during reduction of gold oxide was calculated by integration of the gold oxide reduction peak. The specific charge equivalent of 450 μC cm −2 was used for converting the charge passed during the gold oxide reduction to a total surface area ( A = Q o /450), which was then divided by the mass of the nanoporous gold electrode to obtain a specific surface area per unit mass. Characterization Scanning electron microscopy (SEM) images were obtained with a JEOL 7600F SEM operating at 5 kV in LABE mode. Energy-dispersive X-ray spectroscopy (EDS) was recorded on a JEOL 7600F at 30 kV. TEM images were obtained with a JEM-1400 (JEOL) transmission electron microscope operated at 80 kV. For thin film sectioning, the nanoparticles were first embedded in epoxy resin then sectioned using a Leica Ultramicrotome with diamond knife under cryogenic condition. The 100-nm thin sections were collected and examined using high-resolution TEM (JEOL-2100) at an accelerating voltage of 200 kV. The cross section of the nanoporous gold nanoparticles was also obtained and imaged using FEI Helios Nanolab 600 dual beam focused ion beam/SEM. The sample was precoated with silica as a protective layer against damage of the sample surface by the ion beam. XPS spectra were measured using a Phoibos 100 spectrometer with a monochromatic Mg X-ray radiation source. All XPS spectra were fit using XPS Peak 4.1 (freeware accessible at http://www.phy.cuhk.edu.hk/~surface ). Powder XRD patterns were recorded on a Bruker GADDS XRD diffractometer with Cu K α radiation. How to cite this article : Pedireddy, S. et al. One-step synthesis of zero-dimensional hollow nanoporous gold nanoparticles with enhanced methanol electrooxidation performance. Nat. Commun. 5:4947 doi: 10.1038/ncomms5947 (2014).